A novel phosphor for glareless white light-emitting diodes The luminous efficiency of white light-emitting diodes, which are used as light sources for next-generation illumination, is continuously improving. Presently available white light-emitting diodes emit with extremely high luminance because their emission areas are much smaller than those of conventional light sources. Consequently, white light-emitting diodes produce a glare that is uncomfortable to the human eye. Here we report a yellow-emitting phosphor, the Eu 2+ -doped chlorometasilicate (Ca 1-x-y , Sr x , Eu y ) 7 (SiO 3 ) 6 Cl 2 , which can be used to create glareless white light-emitting diodes. The (Ca 1-x-y , Sr x , Eu y ) 7 (SiO 3 ) 6 Cl 2 exhibits a large Stokes shift, efficiently converting violet excitation light to yellow luminescence, and phosphors based on this host material have much less blue absorption than other phosphors. We used crystal structure analysis to determine the origin of the desired luminescence, and we used (Ca 1-x-y , Sr x , Eu y ) 7 (SiO 3 ) 6 Cl 2 and a blue-emitting phosphor in combination with a violet chip to fabricate glareless white light-emitting diodes that have large emission areas and are suitable for general illumination. Recently, white light-emitting diodes (LEDs) have been receiving attention as light sources because of their energy efficiency [1] , [2] . The major white LEDs presently in the market are phosphor-converted LEDs (pc-LEDs) made of a blue InGaN chip and a yellow phosphor, (Y,Gd) 3 (Al,Ga) 5 O 12 :Ce 3+ (abbreviated YAG:Ce 3+ ) [3] . Its luminescence efficiency exceeds that of fluorescent lamps [4] , [5] . However, as pc-LEDs have much smaller emission areas than conventional light sources, their luminance rises excessively with increasing luminous efficiency, and consequently they produce an uncomfortable glare [6] . The emission areas of pc-LEDs are small, because the yellow-emitting phosphor must be located close to the blue chip to produce a uniform hue; therefore, the phosphor layer is typically deposited on the blue chip so that the chip and the layer have the same geometric area. There have been many reports describing the development of phosphors [7] , [8] , [9] , [10] , [11] , [12] , [13] , [14] , [15] , [16] for violet chips, which have an external quantum efficiency that is intrinsically higher than that of blue chips [17] , [18] , [19] . A pc-LED with a violet chip generates white light only from the luminescence of the phosphors. However, none of the previous reports dealt with glare suppression, which is a major obstacle to the practical application of pc-LEDs. In a pc-LED with a violet chip, two or more phosphors must be mounted on the chip. A combination of blue and yellow phosphors, or a combination of blue, green and red phosphors, is commonly used in pc-LEDs. Glare can be suppressed by expanding the emission area, but such expansion leads to a non-uniform hue. As the green, yellow and red phosphors emit undesirable luminescence by absorbing the light emitted from the blue phosphor [20] , therefore, phosphors that are not excited by the blue light are required. We approached this problem by tuning the excitation properties of the phosphor. In this article, we report a new phosphor, (Ca 1-x-y , Sr x , Eu y ) 7 (SiO 3 ) 6 Cl 2 (abbreviated Cl_MS:Eu 2+ ), which emits yellow luminescence upon violet excitation, with an internal quantum efficiency (IQE) higher than 90% and very weak absorption in the blue wavelength region. These properties allowed us to fabricate a pc-LED composed of a violet chip combined with Cl_MS:Eu 2+ and a blue phosphor, (Ca,Sr) 5 (PO 4 ) 3 Cl:Eu 2+ (APT:Eu 2+ ) [21] . This pc-LED had luminous flux, colour temperature and colour-rendering index values that were adequate for practical use, and it emitted white light with a uniform hue and suppressed glare, thus satisfying the requirements for general illumination. The host, Cl_MS, is a new material with a unique layered structure discovered in this work. Search for a phosphor material In our search for an appropriate phosphor, we explored chemically stable oxide-based materials activated with Eu 2+ , which allows 5 d –4 f transitions. We considered the following features when designing the host material. The primary feature was a mixed-ligand system. In most Eu 2+ oxides, Eu 2+ absorbs in the ultraviolet wavelength region. Shifting the absorption band to the violet region requires a relatively large crystal-field splitting. A strong crystal field is generated when Eu 2+ is located at a site with a distorted co-ordination field [22] , and such a site can be created with a mixed-ligand system. Here we chose oxide and chloride ions as the ligands. The second feature was a layered structure. To obtain a chemically stable phosphor, we chose a host with a layered structure of hydrophilic metal chloride layers alternating with oxide layers. We expected the layering to stabilize the chemically unstable metal chloride layer. As phosphors with layered structures often suffer from substantial thermal quenching of luminescence owing to loose interlayer bonding [23] , [24] , we explored materials that exhibited a small degree of thermal quenching. A survey of materials conducted with these features in mind led us to focus on chlorosilicates [25] , [26] , [27] and ultimately to design a new phosphor material, Cl_MS:Eu 2+ . Crystal structures of Cl_MS and Cl_MS:Eu 2+ We determined the crystal structures of an undoped Cl_MS single crystal and several Eu 2+ -doped powder samples by using synchrotron radiation X-ray diffraction (SR-XRD) at the SPring-8 synchrotron facility in Japan (see Supplementary Methods and Supplementary Tables S1 and S2 ). The structure of Cl_MS:Eu 2+ was found to consist of alternating metal silicate and metal chloride layers along the c axis of a monoclinic unit cell ( Fig. 1a ). The chemical composition of Cl_MS:Eu 2+ was determined to be (Ca 1-x-y , Sr x , Eu y ) 7 (SiO 3 ) 6 Cl 2 (0.167 < x /(1– x – y ) < 2.5; 0.01 < y < 0.3). Cl_MS:Eu 2+ had three cationic sites referred to as M(1), M(2) and M(3), which could accommodate Ca, Sr or Eu. The M(1) site in the metal silicate layer was occupied only by Ca and was co-ordinated by six oxide ions of Si 3 O 9 units [28] to form a [Ca(SiO 3 ) 6 ] framework (see Supplementary Fig. S1 ). The M(2) site was in the metal chloride layer and was occupied by a Sr or Eu ion. This site was co-ordinated by a chloride ion in the metal chloride layer and by seven oxide ions, and thus the site bridged the two metal silicate layers ( Fig. 1b ). The M(3) site at the boundary between the metal silicate and metal chloride layers was occupied by a Ca, Sr or Eu ion, and was co-ordinated by five oxygen ions in the metal silicate layer and by two chloride ions in the metal chloride layer ( Fig. 1b ). We have provided crystal information files in the Supplementary Data Sets 1 and 2 . 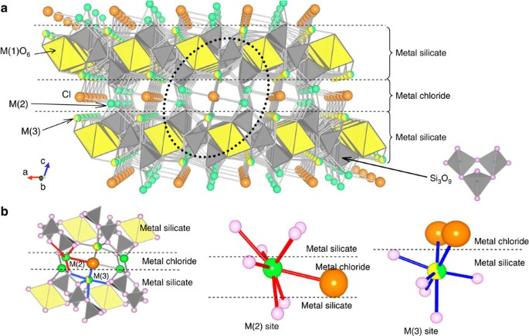Figure 1: Schematic illustration of the crystal structure of (Ca1-x-y,Srx,Euy)7(SiO3)6Cl2. (a) The crystal structure of Cl_MS:Eu2+seen from the b axis. Grey tetrahedra represent SiO4units, yellow octahedra represent M(1)O6units, orange spheres represent chloride ions, green spheres represent M(2) ions, and yellow and green spheres represent M(3) ions. The horizontal dashed lines indicate boundaries between the metal silicate and metal chloride layers. The area indicated by the bold dotted circle is shown in detail inb. The geometry of a Si3O9unit is shown at the lower right of this panel. (b) Detailed illustration of the chemical bonds around the M(2) and M(3) sites. The red and blue sticks indicate chemical bonds between anions and the M(2) and M(3) sites, respectively. Small pink spheres represent oxide ions. The coordination geometries of the M(2) and M(3) sites are also shown separately. Supplementary Data Set 1 includes the crystal structures of an undoped single crystal of Cl_MS at 100 and 300 K. Supplementary Data Set 2 includes the crystal structures of Cl_MS:Eu 2+ at 100 and 300 K. Figure 1: Schematic illustration of the crystal structure of (Ca 1-x-y ,Sr x ,Eu y ) 7 (SiO 3 ) 6 Cl 2 . ( a ) The crystal structure of Cl_MS:Eu 2+ seen from the b axis. Grey tetrahedra represent SiO 4 units, yellow octahedra represent M(1)O 6 units, orange spheres represent chloride ions, green spheres represent M(2) ions, and yellow and green spheres represent M(3) ions. The horizontal dashed lines indicate boundaries between the metal silicate and metal chloride layers. The area indicated by the bold dotted circle is shown in detail in b . The geometry of a Si 3 O 9 unit is shown at the lower right of this panel. ( b ) Detailed illustration of the chemical bonds around the M(2) and M(3) sites. The red and blue sticks indicate chemical bonds between anions and the M(2) and M(3) sites, respectively. Small pink spheres represent oxide ions. The coordination geometries of the M(2) and M(3) sites are also shown separately. Full size image Luminescence spectrum of Cl_MS:Eu 2+ The luminescence spectrum of (Ca 0.37 Sr 0.53 Eu 0.10 ) 7 (SiO 3 ) 6 Cl 2 obtained with a 400-nm excitation at room temperature exhibited a single band at 580 nm, with a full width at half-maximum of 3.6×10 3 cm −1 ( Fig. 2a ). The corresponding excitation spectrum exhibited strong absorption at wavelengths of 410 nm or shorter, but the intensity of the absorption rapidly decreased at wavelengths longer than 420 nm. Consequently, an ~450-nm blue light was only weakly absorbed by Cl_MS:Eu 2+ . Thus, the excitation spectrum of Cl_MS:Eu 2+ distinctly differed from the excitation spectra of other phosphors used for violet excitation. For example, the excitation spectra of (Ba,Sr) 2 SiO 4 :Eu 2+ (ref. 29 ) and (Sr,Ca)AlSiN 3 :Eu 2+ (refs 30 , 31 ) exhibit considerable absorption intensity around 450 nm ( Fig. 2a ). In addition, the magnitude of the Stokes shift (ΔS) for Cl_MS:Eu 2+ was 6.9×10 3 cm −1 , which was much larger than that observed for conventional phosphors ( Fig. 2a ). The emission colour of Cl_MS:Eu 2+ could be tuned by varying the Ca/Sr atomic ratio. We examined the Ca fraction dependence of the dominant wavelength (that is, the wavelength of monochromatic light that was the same colour as the band luminescence), and found that as the Ca/Sr ratio was increased the dominant wavelength was linearly red-shifted ( Fig. 2b ). The IQEs and absorptions at the dominant wavelength were almost equivalent. The luminescence spectra of typical samples are shown in Supplementary Fig. S2 . The luminescence intensity of Cl_MS:Eu 2+ was stable to Eu 2+ concentration and temperature. Even though the Eu 2+ concentration in Cl_MS:Eu 2+ increased by more than 20 atom%, the samples consisted almost completely of a single phase that contained only a few impurities (see Supplementary Fig. S3 ). No concentration quenching occurred at Eu 2+ concentrations up to 20 atom% ( Fig. 2c and Supplementary Table S3 ). The highest luminescence intensity was observed at a dopant level of 10 atom%, (Ca 0.37 Sr 0.53 Eu 0.10 ) 7 (SiO 3 ) 6 Cl 2 , and the IQE and the absorption were 94% and 90%, respectively, upon excitation by a 407-nm laser diode. A luminescence intensity of 75% relative to the room temperature value was observed at 423 K ( Fig. 2d ). This temperature dependence was comparable to that of YAG:Ce 3+ . A life test in air at 85% humidity and 358 K showed that the variation in luminescence intensity was within 2% after 2,000 h; this variation was less than the variation observed for (Ba,Sr) 2 SiO 4 :Eu 2+ after only 500 h of testing ( Fig. 2e ). 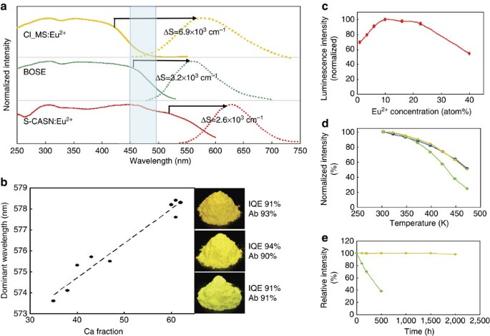Figure 2: Luminescence properties of Cl_MS:Eu2+. (a) Luminescence (dotted curves) and excitation spectra (solid curves) of phosphors with excitation at 400 nm and monitoring at 580 nm. The yellow curves show spectra of (Ca0.37Sr0.53Eu0.10)7(SiO3)6Cl2. For comparison, the spectra of two conventional phosphors are also shown; (Ba,Sr)2SiO4:Eu2+(BOSE; green curves; excitation at 400 nm; monitoring at 560 nm) and (Sr,Ca)AlSiN3:Eu2+(S-CASN:Eu2+; red curves; excitation at 400 nm; monitoring at 630 nm). The area hatched in blue indicates the wavelengths of blue light. The Stokes shift values (ΔS) are also shown. (b) Dominant wavelength of luminescence as a function of Ca fraction in Cl_MS:Eu2+. The IQE and absorption (Ab) values for Cl_MS:Eu2+samples with luminescence at various dominant wavelengths are also shown. (c) Normalized luminescence intensity for the 400-nm excitation of Cl_MS:Eu2+as a function of Eu2+concentration. (d) Temperature dependence of luminescence intensity normalized to intensity at 303 K. The yellow, blue and green curves indicate Cl_MS:Eu2+, YAG:Ce3+and BOSE, respectively. (e) Relative luminescence intensity as a function of time at 358 K and 85% humidity. The yellow and green curves indicate Cl_MS:Eu2+and BOSE, respectively. Figure 2: Luminescence properties of Cl_MS:Eu 2+ . ( a ) Luminescence (dotted curves) and excitation spectra (solid curves) of phosphors with excitation at 400 nm and monitoring at 580 nm. The yellow curves show spectra of (Ca 0.37 Sr 0.53 Eu 0.10 ) 7 (SiO 3 ) 6 Cl 2 . For comparison, the spectra of two conventional phosphors are also shown; (Ba,Sr) 2 SiO 4 :Eu 2+ (BOSE; green curves; excitation at 400 nm; monitoring at 560 nm) and (Sr,Ca)AlSiN 3 :Eu 2+ (S-CASN:Eu 2+ ; red curves; excitation at 400 nm; monitoring at 630 nm). The area hatched in blue indicates the wavelengths of blue light. The Stokes shift values (ΔS) are also shown. ( b ) Dominant wavelength of luminescence as a function of Ca fraction in Cl_MS:Eu 2+ . The IQE and absorption (Ab) values for Cl_MS:Eu 2+ samples with luminescence at various dominant wavelengths are also shown. ( c ) Normalized luminescence intensity for the 400-nm excitation of Cl_MS:Eu 2+ as a function of Eu 2+ concentration. ( d ) Temperature dependence of luminescence intensity normalized to intensity at 303 K. The yellow, blue and green curves indicate Cl_MS:Eu 2+ , YAG:Ce 3+ and BOSE, respectively. ( e ) Relative luminescence intensity as a function of time at 358 K and 85% humidity. The yellow and green curves indicate Cl_MS:Eu 2+ and BOSE, respectively. Full size image Eu 2+ sites of Cl_MS:Eu 2+ Upon excitation with ultraviolet radiation ( Fig. 3a ), a peak at 480 nm appeared in the luminescence spectrum of (Ca 0.40 Sr 0.56 Eu 0.04 ) 7 (SiO 3 ) 6 Cl 2 . The excitation spectrum of this emission band (480 nm) differed from that monitored at 580 nm; the former spectrum exhibited a narrow band peaking at 310 nm with weak violet absorption. This result confirmed that Cl_MS:Eu 2+ had two different Eu 2+ -occupied sites, the M(2) and M(3) sites ( Fig. 1b ). To clarify the correspondence between the two crystallographic sites and the emission bands, we investigated the temperature dependence of the luminescence intensity and of the crystal structure. We plotted the radiative decay curves for (Ca 0.40 Sr 0.56 Eu 0.04 ) 7 (SiO 3 ) 6 Cl 2 at 100 and 300 K upon excitation with a 266-nm laser pulse with monitoring at 480 and 580 nm ( Fig. 3b,c ). All the decay curves consisted of fast and slow components (with lifetimes τ 1 and τ 2 , respectively), and were fitted by double exponential components. Here we discuss the fast component of each decay curve. The shorter lifetime of the 480-nm band ( τ 1 ) showed large temperature dependence between 100 and 300 K, whereas neither τ 1 nor τ 2 of the 580-nm band changed substantially with temperature. The SR-XRD analysis ( Fig. 3d ) revealed that the local structure of the M(2) site changed markedly with increasing temperature; three of the seven M(2)–O bonds lengthened by more than 0.02 Å. In contrast, the bond lengths at the M(3) site did not change markedly with increasing temperature ( Fig. 3d ). Consequently, we attributed the 580-nm band to Eu 2+ at the M(3) site and the 480-nm band to Eu 2+ at the M(2) site. 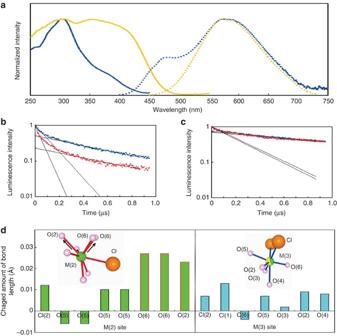Figure 3: Temperature dependence of the luminescence properties and bond lengths of (Ca0.40Sr0.56Eu0.04)7(SiO3)6Cl2. (a) Room temperature luminescence spectra with excitation at 310 (dotted blue curve) and 400 nm (dotted yellow curve), and excitation spectra monitored at 480 (solid blue curve) and 580 nm (solid yellow curve). (b) Radiative decay curves of Eu2+luminescence at 480 nm. Blue and red lines indicate data measured at 100 and 300 K, respectively. Both decay curves consisted of fast and slow components. The lifetime (τ1) of the fast component was 0.12 μs at 100 K and 0.06 μs at 300 K. The lifetime (τ2) of the slow component was 0.62 μs at 100 K and 0.63 μs at 300 K. (c) Radiative decay curves of Eu2+luminescence at 580 nm. Blue and red lines indicate data measured at 100 and 300 K, respectively. Both decay curves consisted of fast and slow components. The lifetime (τ1) of the fast component was 0.26 μs at 100 K and 0.27 μs at 300 K. The lifetime (τ2) of the slow component was 1.4 μs at 100 K and 1.4 μs at 300 K. (d) Difference of the bond distances at 100 and 300 K for the M(2) and M(3) sites, as indicated by SR-XRD data. Positive values indicate bond elongation, and negative values indicate bond shortening with increasing temperature. Figure 3: Temperature dependence of the luminescence properties and bond lengths of (Ca 0.40 Sr 0.56 Eu 0.04 ) 7 (SiO 3 ) 6 Cl 2 . ( a ) Room temperature luminescence spectra with excitation at 310 (dotted blue curve) and 400 nm (dotted yellow curve), and excitation spectra monitored at 480 (solid blue curve) and 580 nm (solid yellow curve). ( b ) Radiative decay curves of Eu 2+ luminescence at 480 nm. Blue and red lines indicate data measured at 100 and 300 K, respectively. Both decay curves consisted of fast and slow components. The lifetime ( τ 1 ) of the fast component was 0.12 μs at 100 K and 0.06 μs at 300 K. The lifetime ( τ 2 ) of the slow component was 0.62 μs at 100 K and 0.63 μs at 300 K. ( c ) Radiative decay curves of Eu 2+ luminescence at 580 nm. Blue and red lines indicate data measured at 100 and 300 K, respectively. Both decay curves consisted of fast and slow components. The lifetime ( τ 1 ) of the fast component was 0.26 μs at 100 K and 0.27 μs at 300 K. The lifetime ( τ 2 ) of the slow component was 1.4 μs at 100 K and 1.4 μs at 300 K. ( d ) Difference of the bond distances at 100 and 300 K for the M(2) and M(3) sites, as indicated by SR-XRD data. Positive values indicate bond elongation, and negative values indicate bond shortening with increasing temperature. Full size image The M(3)-site Eu 2+ ion, which gave rise to the 580-nm band, was co-ordinated by the mixed ligand, that is, a single bridging oxygen ion, four non-bridging oxygen ions and two chloride ions ( Fig. 1b ), and was located at the boundary between the metal silicate and metal chloride layers. The asymmetric coordination structure of the M(3) site resulted in a large crystal-field splitting and an absorption band at a wavelength in the violet region, but not extending to the blue region. We evaluated the asymmetry of the Eu 2+ sites by calculating electrical field gradients (EFGs) for the M(2) and M(3) sites using density functional theory (DFT). The initial structural parameters were taken from single-crystal SR-XRD data for CaSr 2 (Ca 0.55 Sr 0.45 ) 4 Si 6 O 18 Cl 2 at 100 K. In the calculation, we modelled the mixed occupation of the M(3) sites with Ca and Sr by the ordered structure shown in Supplementary Fig. S4 . To obtain a relaxed structure, we optimized the geometry with the Vienna Ab Initio Simulation Package code [32] using the projected, augmented plane-wave method [33] . The EFG parameters were calculated with the WIEN2k programme package [34] , which adopts a full-potential, all-electron method that utilizes the full-potential, linearized, augmented plane-wave+local orbitals approach [35] . In each calculation procedure, the exchange and correlation potentials within the DFT were calculated with the Perdew–Burke–Ernzerhof generalized gradient approximation [36] . The principal axes of the EFG tensors of the Sr 2+ and Ca 2+ ions at the M(2) and M(3) sites, respectively, are illustrated schematically in Fig. 4a , and the EFG tensor elements at the M(2) and M(3) sites calculated by DFT are summarized in Table 1 . The asymmetry parameters η of the M(2) and M(3) sites could be derived by using the EFG tensor elements (defined at the bottom of Table 1 ). The value of η at the M(3) site was clearly much higher than that at the M(2) site. 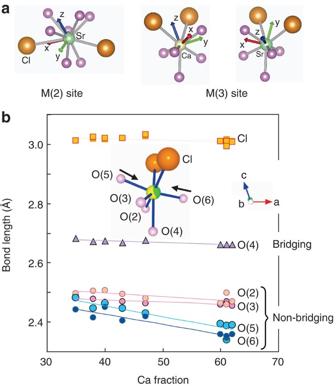Figure 4: Local structure of Eu2+occupancy sites of Cl_MS:Eu2+. (a) Schematic illustrations of principal axes of EFG tensors of Sr2+and Ca2+ions at the M(2) and M(3) sites. (b) Effect of Ca fraction on M(3)–anion bond distance at the M(3) site, as indicated by SR-XRD data: M(3)–Cl (orange squares); M(3)–O(4) (violet triangles; O(4) is a bridging oxygen); and M(3)–O(2), –O(3), –O(5) and –O(6) (pink and blue circles; these are non-bridging oxygens). Figure 4: Local structure of Eu 2+ occupancy sites of Cl_MS:Eu 2+ . ( a ) Schematic illustrations of principal axes of EFG tensors of Sr 2+ and Ca 2+ ions at the M(2) and M(3) sites. ( b ) Effect of Ca fraction on M(3)–anion bond distance at the M(3) site, as indicated by SR-XRD data: M(3)–Cl (orange squares); M(3)–O(4) (violet triangles; O(4) is a bridging oxygen); and M(3)–O(2), –O(3), –O(5) and –O(6) (pink and blue circles; these are non-bridging oxygens). Full size image Table 1 EFG tensor elements ( V xx , V yy , V zz ) and asymmetric parameter η from DFT calculations. Full size table The changes in the local structure of the M(3) site due to the increase in the Ca fraction induced a red shift of the luminescence. Anisotropic lattice contraction occurred along the a axis (see Supplementary Fig. S5 ), owing to shortening of the O(5)–M(3)–O(6) bonds with increasing Ca fraction ( Fig. 4b ). This contraction induced substantial deformation around the M(3) site. As such deformation widened the crystal-field splitting, the 580-nm luminescence band was red-shifted by a reduction of the lowest 5 d energy level. These results are consistent with the calculated results, indicating that the η value for Ca at the M(3) site was larger than that for Sr ( Table 1 ). Cl_MS:Eu 2+ exhibited a high IQE. IQE is given by Yamamoto [37] where W is the luminescence radiation probability and N is the non-radiative transition probability. The main factors that affect the non-radiative transition probability are thermal quenching and concentration quenching. The IQE of Cl_MS:Eu 2+ was very high because the influence of these factors was small owing to the following reasons. Thermal expansion of Cl_MS:Eu 2+ was anisotropic. The lattice constants increased linearly with increasing temperature from 100 to 573 K as shown in Supplementary Fig. S6 . The linear thermal expansion co-efficient along the c axis, the direction perpendicular to the layers, was larger than that along the a- and b axes. The values along the c-, a- and b axes at 300 K were 1.8×10 5 , 5.4×10 6 and 7.5×10 6 K −1 , respectively. At the M(2) site, which bridged the metal silicate layers, the cation–oxygen bond lengths were markedly increased by thermal expansion of the interlayer separation. These lengthened bonds resulted in a shorter luminescence lifetime for the 480-nm band. In contrast, the change in the Eu 2+ –anion distance was less at the M(3) site, which had few co-ordinated oxide ions in the stacked-layer direction. Consequently, thermal quenching of the 580-nm band was sufficiently small for practical applications, despite the material's layered structure. Concentration quenching of the main emission band (the 580-nm band) of Cl_MS:Eu 2+ was not observed ( Fig. 2c ), but the 480-nm band was drastically affected by concentration quenching (see Supplementary Fig. S7 ). We cannot explain, on the basis of the experimental results, why concentration quenching of the M(3) site did not occur. The conspicuous difference in the sensitivity of the M(2) and M(3) sites to concentration quenching appears to have to do with local asymmetry around each site, which controlled the energy transfer processes from the excited Eu 2+ . There have been reports indicating that phosphors with a low-dimensional arrangement of the dopant ions show little concentration quenching [38] . In such phosphors, the stoichiometric phosphors (100% dopant ion) are also contained [39] , [40] . The dopant ion site of these phosphors has higher asymmetry, owing to low-dimensional arrangement. This observation is consistent with the fact that the M(3) site, which had lower symmetry and a low-dimensional arrangement, did not exhibit concentration quenching. To evaluate the practical applicability of the Cl_MS:Eu 2+ phosphor, we fabricated three sample pc-LEDs consisting of a violet or blue chip encapsulated in translucent resin containing various phosphors ( Fig. 5a ). Sample 1 was prepared with a violet chip coupled with (Ca 0.37 Sr 0.53 Eu 0.10 ) 7 (SiO 3 ) 6 Cl 2 and the blue phosphor APT:Eu 2+ ( Fig. 5b ). For reference, we also prepared pc-LEDs of the same structure with a blue chip coupled with YAG:Ce 3+ (sample 2, Fig. 5c ) and with a violet chip coupled with three primary-colour phosphors (sample 3, Fig. 5d ). The differences in the emission colour distribution in the emission area of these three samples were measured with a two-dimensional colour analyser ( Fig. 5e,f,g ). Sample 1 exhibited a uniform hue over the entire resin dome, similar to that of an incandescent lamp, but samples 2 and 3 showed red-shifted colour on the rim of the dome, resulting in a non-uniform hue. The performance of these three samples is summarized in Supplementary Table S4 . 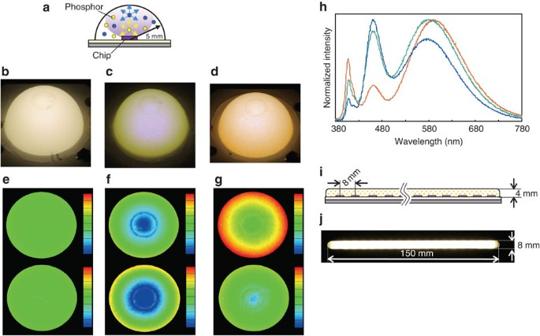Figure 5: Structure and performance of fabricated pc-LEDs. (a) Structure of fabricated pc-LEDs. (b–d) Images of emitting fabricated pc-LEDs with different phosphors and chips. Sample 1 consists of (Ca0.37Sr0.53Eu0.10)7(SiO3)6Cl2and APT:Eu2+coupled with a violet chip (λp=405 nm) inb; sample 2 consists of YAG:Ce3+coupled with a blue chip (λp=460 nm) inc; and sample 3 consists of a mixture of APT:Eu2+, β-SiAlON:Eu2+and S-CASN:Eu2+coupled with a violet chip (λp=405 nm) ind. (e–g) Emission colour distribution in emission areas of sample 1 ine, sample 2 infand sample 3 ing. The upper pictures show the distribution ofCxvalues used for Commission Internationale de l'Eclairage chromaticity, and the lower pictures are theCyvalues. The scale bars forCxrepresent the same chromaticity range in all the panels. The minimum (blue) value is 0.277, and the maximum (red) value is 0.443. The scale bars forCyrepresent the same chromaticity range in all the panels. The minimum (blue) value is 0.294, and the maximum (red) value is 0.460. The operation current was 350 mA. (h) Luminescence spectra of Cl_MS:Eu2+pc-LEDs with different colour temperatures, operated at 350 mA. The orange curve indicates 3,010 K , the green curve 4,100 K and the blue curve 5,070 K. (i) Schematic illustration of a line-shaped module. (j) Image of the emitting line-shaped module. Figure 5: Structure and performance of fabricated pc-LEDs. ( a ) Structure of fabricated pc-LEDs. ( b–d ) Images of emitting fabricated pc-LEDs with different phosphors and chips. Sample 1 consists of (Ca 0.37 Sr 0.53 Eu 0.10 ) 7 (SiO 3 ) 6 Cl 2 and APT:Eu 2+ coupled with a violet chip ( λ p =405 nm) in b ; sample 2 consists of YAG:Ce 3+ coupled with a blue chip ( λ p =460 nm) in c ; and sample 3 consists of a mixture of APT:Eu 2+ , β-SiAlON:Eu 2+ and S-CASN:Eu 2+ coupled with a violet chip (λ p =405 nm) in d . ( e–g ) Emission colour distribution in emission areas of sample 1 in e , sample 2 in f and sample 3 in g . The upper pictures show the distribution of C x values used for Commission Internationale de l'Eclairage chromaticity, and the lower pictures are the C y values. The scale bars for C x represent the same chromaticity range in all the panels. The minimum (blue) value is 0.277, and the maximum (red) value is 0.443. The scale bars for C y represent the same chromaticity range in all the panels. The minimum (blue) value is 0.294, and the maximum (red) value is 0.460. The operation current was 350 mA. ( h ) Luminescence spectra of Cl_MS:Eu 2+ pc-LEDs with different colour temperatures, operated at 350 mA. The orange curve indicates 3,010 K , the green curve 4,100 K and the blue curve 5,070 K. ( i ) Schematic illustration of a line-shaped module. ( j ) Image of the emitting line-shaped module. Full size image Sample 1 exhibited a luminous flux of 88 lm and a luminance of 1.0 cd mm −2 at an operating current of 350 mA. For comparison, a surface-mount device (SMD) pc-LED, which is a commonly used type of pc-LED, exhibited a luminous flux of 85 lm and a luminance of 11 cd mm −2 . The SMD pc-LED consisted of a thin phosphor layer deposited on a chip mounted at the bottom of a small casing (see Supplementary Fig. S8 ). The unified glare rating (UGR), which is used to evaluate glare, is given by the CIE [41] where L b is the background luminance (cd m −2 ), L is the source luminance (cd m −2 ), ω is the solid angle of the source (sr) and p is the position index (the positional relationship between the light source and the line of sight). The form of this equation indicates that as the source luminance increases, UGR rises and glare becomes uncomfortable. In sample 1, the luminance was reduced to less than 1/10 of that for the SMD pc-LED without a decrease in luminous flux; thus, unwanted glare was suppressed (see Supplementary Methods and Supplementary Fig. S9 ). After continuous operation at 350 mA for 3,000 h, the luminous flux of sample 1 was still at least 96% of its initial value. The colour temperature was 4,100 K for sample 1, and the temperature could be tuned from 3,010 to 5,070 K by varying the Ca fraction ( Fig. 5h ). We also fabricated a line-shaped module consisting of a row of pc-LEDs fabricated with Cl_MS:Eu 2+ ( Fig 5i,j ). The module contained 18 violet chips aligned with a pitch of 8 mm. The chips were encapsulated thickly in a semi-cylindrical form, with resin containing Cl_MS:Eu 2+ phosphors. White-light emission from this device was uniform in hue over an area of 150×8 mm 2 , and the module exhibited a luminous flux of 500 lm with a luminous efficiency of 90 lm W −1 . In conclusion, we have developed a phosphor for a violet chip, Cl_MS:Eu 2+ , based on a newly discovered host crystal with a mixed-ligand system and a layered structure. Cl_MS:Eu 2+ exhibited a large Stokes shift, efficiently converting violet light to yellow luminescence, and the luminous efficiency showed good temperature dependence despite the material's layered structure. The use of Cl_MS:Eu 2+ in conjunction with violet LED chips allowed us to fabricate glareless pc-LEDs suitable for general illumination with uniform hue, moderate luminance, adequate colour-rendering index and high luminous flux. Furthermore, pc-LEDs prepared with Cl_MS:Eu 2+ can be expected to permit the fabrication of light sources with new shapes, such as domes or elongated semicylinders. Sample preparation Single crystals of undoped Cl_MS were grown by the self-flux method, in which SrCl 2 acted as both a starting material and a flux. For the formation of a sufficient quantity of liquid flux, SrCl 2 was added in excess (7.5 times the stoichiometric amount). The other starting material, SiO 2 , was also added in excess (1.2 times the stoichiometric amount) because it is not very reactive. SrCl 2 , SiO 2 and a stoichiometric amount of CaCO 3 , all of 3N or higher purity, were thoroughly mixed and pelletized. The pellets were heated at 1,030 °C for 36 h in air and then cooled to room temperature at a rate of 300 °C h −1 . The resulting Cl_MS crystals were collected by washing off the remaining flux with warm water. We prepared samples of Eu 2+ -doped Cl_MS by using the method described for Cl_MS, with Eu 2 O 3 or EuCl 3 as the Eu source. The Eu 2+ fraction per divalent metal ion was 3–50 atom%. The pellets were fired at 1,030 °C for 10 h in a reducing atmosphere of H 2 /N 2 (5/95). Fabrication of pc-LEDs Phosphors of different emission colours were mixed at the following weight ratios to provide white emission of specified colour coordinates: Cl_MS:Eu 2+ /APT:Eu 2+ =1.8/1.0 for pc-LED sample 1, 100% YAG:Ce 3+ for pc-LED sample 2 and (Sr,Ca)AlSiN 3 :Eu 2+ /β-SiAlON/APT:Eu 2+ =0.6/1.1/1.0 for pc-LED sample 3. Then a phosphor paste was made by dispersion of each of the above phosphor mixtures in translucent silicone resin at a concentration of 0.2–1.3 vol%. Finally, a pc-LED was fabricated by encapsulation of an LED chip on a white substrate with the phosphor paste, which was allowed to harden at 150 °C for 90 min. Determination of crystal structures SR-XRD measurements were performed at the Japan Synchrotron Radiation Research Institute, SPring-8, with synchrotron orbit radiation on the BL02B1 and BL02B2 beamlines at a wavelength of ca. 0.35 Å for the single crystals and a wavelength of ca. 0.80 Å for the Eu 2+ -doped powder samples. The initial atomic positions of Cl_MS were determined directly from the data for the undoped single crystal (see Supplementary Methods ). Optical measurements The luminescence spectra under continuous excitation and the excitation spectra of the phosphor samples were measured at room temperature with a multichannel optical analyser (PMA C5966-31, Hamamatsu Photonics). Time-resolved luminescence spectra were measured with a pulsed 266-nm laser (CFR 400, Quantel), with an excitation duration of 10 ns and a repetition rate of 10 Hz. IQEs and absorptions were obtained from luminescence spectra with 407-nm laser-diode excitation, using a phosphor sample mounted in an integrated sphere. The detector employed a spectrometer (CAS 140B-152, Instrument Systems). This measurement system had two key features. First, the energy density of the excitation beam with which the sample was irradiated was high. The energy density was as high as actually mounted on an LED chip. Second, the measurement time was short, because a charge-coupled device (CCD) image sensor array was used as a detector. Consequently, we could measure the IQEs without the influence of thermal quenching by the Stokes shift. The integrating sphere had a diameter of 150 mm and three ports with diameters of 25 mm. The sample was placed in the integrating sphere through the bottom port, and excitation light was directed onto the sample from the upper port. Emitted light was directed to the spectrometer through an optical receiver installed in the middle port. We obtained data by gathering the reflections generated by irradiation of the sample with a laser-diode beam (power, 10.2 mW at 407 nm; irradiation time, 10 ms; irradiated area, 1 mm diameter). The detector of the CAS 140B-152 spectrometer was the CCD array, which has 1,024 CCD elements. The wavelength band that could be measured was between 375–785 nm. The reflection spectrum of the BaSO 4 powder without absorption was used as a reference for calculation of the IQE and the absorption. The CAS 140B-152 spectrometer was also used to obtain luminous flux, colour coordinates and colour temperature from a pc-LED operated in an integrated sphere. A two-dimensional colour analyser (CM-1500M, Minolta) was used to obtain the luminance and emission colour distribution on the pc-LEDs. How to cite this article: Daicho, H. et al . A novel phosphor for glareless white light-emitting diodes. Nat. Commun. 3:1132 doi: 10.1038/ncomms2138 (2012).